Extracellular palladium-catalysed dealkylation of 5-fluoro-1-propargyl-uracil as a bioorthogonally activated prodrug approach A bioorthogonal organometallic reaction is a biocompatible transformation undergone by a synthetic material exclusively through the mediation of a non-biotic metal source; a selective process used to label biomolecules and activate probes in biological environs. Here we report the in vitro bioorthogonal generation of 5-fluorouracil from a biologically inert precursor by heterogeneous Pd 0 catalysis. Although independently harmless, combined treatment of 5-fluoro-1-propargyl-uracil and Pd 0 -functionalized resins exhibits comparable antiproliferative properties to the unmodified drug in colorectal and pancreatic cancer cells. Live-cell imaging and immunoassay studies demonstrate that the cytotoxic activity of the prodrug/Pd 0 -resin combination is due to the in situ generation of 5-fluorouracil. Pd 0 -resins can be carefully implanted in the yolk sac of zebrafish embryos and display excellent biocompatibility and local catalytic activity. The in vitro efficacy shown by this masking/activation strategy underlines its potential to develop a bioorthogonally activated prodrug approach and supports further in vivo investigations. Bertozzi’s landmark works in the early 2000s (refs 1 , 2 ) demonstrated that artificial chemistry and biological chemistry can take place within the same physical space, yet do not interfere with each other. Through the development of labelling strategies based on the chemospecific conjugation of two biologically-inert reactive partners, this revolutionary chemical paradigm—so-called bioorthogonal chemistry—has enabled the non-intrusive real-time study of a wide range of biomolecules in their native environs [3] , [4] . Because of the exclusive nature of the bioorthogonal concept, the range of chemical reactions that meets its requirements has been limited in practice to the Staudinger ligation [1] and cycloadditions between spring-loaded reactive partners (metal-free click chemistry [2] , [3] , [4] ). Nevertheless, the bioorthogonal concept may integrate additional bio-independent chemical processes that are promoted by abiotic activators such as biocompatible electromagnetic radiations [5] , [6] , [7] and non-biological transition metals [8] , [9] . Although the application of transition metals in medicine have been investigated for many centuries, its use to mediate chemoselective transformations in cells—for example, bioorthogonal organometallic (BOOM) reactions [8] —is a recent addition to the chemical biology field [8] , [9] , [10] , [11] , [12] , [13] , [14] . In 2006, Streu and Meggers [10] described the first application of a ruthenium catalyst to carry out Alloc deprotection of a caged fluorophore inside human cells. The aim to minimize the inherent toxicity of the catalyst motivated the Bradley group to investigate heterogeneous catalysis to mediate palladium chemistry inside cells. Pd 0 -functionalized microspheres operated as a dual catalytic/cell delivery system able to enter cells in vitro and catalyse allylcarbamate cleavage and Suzuki-Miyaura cross-coupling in the cytoplasm without cytotoxicity [9] , [11] . Notable examples of palladium-based applications in cell culture includes copper-free Sonogashira coupling of an alkyne-encoded cytoplasmic ubiquitin protein [12] , extracellular Suzuki reaction to label Escherichia coli cell surface components [13] and the detection of intracellular CO based on the reactivity of a cyclopalladated probe towards carbonylation [14] . Owing to its biological inertness, metallic Pd 0 shows the safest toxicity profile among all palladium species [15] and is frequently used in metal alloys for dental restoration [16] . Based on the unique catalytic properties and biocompatibility of this metal, we hypothesized that extracellular heterogeneous catalysis mediated by a palladium-functionalized implant could enable the chemospecific conversion of a systemically administered prodrug into its active form in a spatially controlled manner. As opposed to biolabile prodrugs, whose activation process relies on metabolic pathways [17] , an efficient palladium-activated prodrug therapy would be entirely dependent on the distinct catalytic properties of this transition metal and therefore the prodrug would remain intact in the absence of a palladium source. By intratumoural implantation of a metal-functionalized device, palladium-labile prodrugs would be exclusively activated within the cancerous tissue. Locoregional generation of cytotoxic agents would enable increasing dosing while reducing adverse side effects in distant tissues and organs, an optimal strategy to treat advanced tumours that cannot be resected by surgery. Notably, this spatially targeted approach would serve to expand the therapeutic window and scope of potent cytotoxic drugs such as 5-fluorouracil (5FU), which has a long history in oncology practice but a clinical activity limited by its safety profile [18] . 5FU is converted intracellularly into cytotoxic nucleotidic metabolites via functionalization on its N 1 position. Its active metabolites either inhibit directly thymidylate synthase or become incorporated into RNA and DNA molecules to disrupt normal cell functions ( Fig. 1 ) [19] . Based on this mode of action, modification of the N 1 position of 5FU with biochemically stable groups would hinder its intracellular activation and result in a significant loss of cytotoxic activity. Here we report the introduction of allyl, propargyl and benzyl moieties at the N 1 position of 5FU as a means to minimize prodrug’s susceptibility to cleavage by hydrolytic enzymes, while, at the same time, rendering them potentially sensitive to palladium catalysis. These alkyl functional groups have been widely used in organic synthesis as OH protection strategies [20] and, importantly, recent studies have shown the sensitivity of allyl and propargyl phenolic ethers to oxidative cleavage by palladium species in biocompatible conditions [21] , [22] , [23] . Although palladium-mediated N -dealkylations typically require temperatures incompatible with cell survival (>80 °C) [24] , [25] , [26] , we hypothesized that the particular features of the 5FU heterocyclic system (relatively low p K a values because of the charge delocalization of 5FU aromatic conjugate bases [27] , Supplementary Fig. 1a ) could promote its properties as a leaving group relative to more basic amino groups. 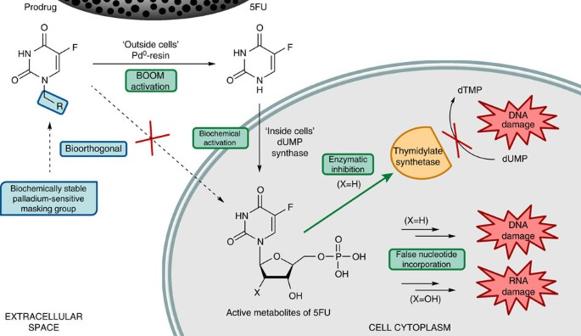Figure 1: Bioorthogonally activated prodrug strategy and toxigenic mode of action. Chemical masking of theN1 position of 5-fluorouracil (5FU) with a biochemically inert palladium-sensitive group would impede 5FU intracellular activation and, consequently, prevent its pharmacological activity. Such a prodrug will be selectively converted into 5FU by the catalysis of Pd0, for instance, in the affected area, organ or tissue where a Pd0-functionalized device has been surgically implanted, thus inducing a local treatment of the disease and reducing side effects of drug in distant tissues and organs. dTMP, thymidine monophosphate; dUMP, deoxyuridine monophosphate. Figure 1: Bioorthogonally activated prodrug strategy and toxigenic mode of action. Chemical masking of the N 1 position of 5-fluorouracil (5FU) with a biochemically inert palladium-sensitive group would impede 5FU intracellular activation and, consequently, prevent its pharmacological activity. Such a prodrug will be selectively converted into 5FU by the catalysis of Pd 0 , for instance, in the affected area, organ or tissue where a Pd 0 -functionalized device has been surgically implanted, thus inducing a local treatment of the disease and reducing side effects of drug in distant tissues and organs. dTMP, thymidine monophosphate; dUMP, deoxyuridine monophosphate. Full size image To activate prodrugs in the extracellular space, we investigate the application of a robust heterogeneous catalytic system based on Pd 0 -functionalized polyethylene glycol (PEG)-polystyrene resins [28] (Pd 0 -resins) that are larger than human cells (150 μm in diameter). As previously reported [9] , [11] , Pd 0 nanoparticles display high catalytic activity, can be readily generated and trapped in an amino-functionalized polymer matrix, and are safe for biological applications. Our results show that alkylation of the N 1 position of 5FU suppresses the drug’s cytotoxic properties and exhibits full stability in cell culture. Remarkably, the propargyl derivative (5-fluoro-1-propargyl-uracil ( Pro-5FU )) displays high sensitivity to Pd 0 -mediated heterogeneous catalysis, thus allowing the bioorthogonal generation of 5FU under biocompatible conditions (37 °C, isotonic media and physiologic pH). Although independently harmless, combined treatment of Pro-5FU and Pd 0 -resins exhibits equivalent antiproliferative properties to unmodified 5FU in colorectal and pancreatic cancer cells, underlining the in vitro efficacy of this unprecedented masking/activation strategy. Preparation of Pd 0 -resins and 5FU prodrugs Pd 0 -resins ( Fig. 2a,b ) were prepared from NovaSyn TG amino resin HL using the procedure developed in the Bradley group [28] with minor modifications. Transmission electron microscope images showed dark nanoparticles (5 nm) regularly distributed across the resins ( Fig. 2b ), whereas the powder X-ray diffraction spectra presented the distinctive pattern of the face-centred cubic lattice of Pd 0 ( Supplementary Fig. 1b ). Pd 0 -resins were visibly differentiated from non-functionalized resins (naked resins) because of the dark colour of the former ( Supplementary Fig. 1c ). Palladium content was determined to be 2.83% (w/w) by inductively coupled plasma-optical emission spectrometry. 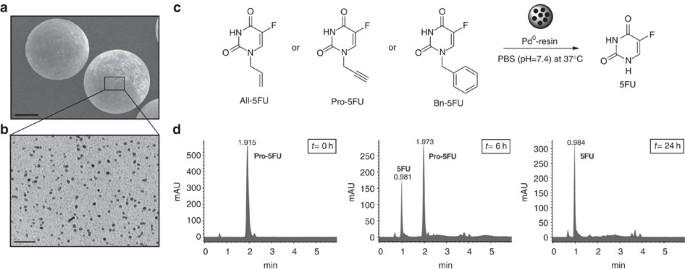Figure 2: Pd0-mediated prodrug-into-drug conversion assays in biocompatible environment. (a) Scanning electron microscope image of Pd0-resins at approximately 200 magnification. Scale bar, 50 μm. (b) Transmission electron microscope image of a Pd0-resin cross-section at approximately 190,000 magnification. Scale bar, 50 nm. (c) Pd0-mediated dealkylation of 5-fluorouracil (5FU) prodrugs under biocompatible conditions (37 °C, isotonic media and physiologic pH). (d) Representative HPLC traces of Pd0-mediated conversion ofPro-5FUinto 5FU. Reaction crudes were analysed using an ultraviolet detector (280 nm) att=0 h,t=6 h andt=24 h. Conversion studies were performed in triplicate.All-5FU, 1-allyl-5FU;Bn-5FU, 1-benzyl-5FU;Pro-5FU, 5-fluoro-1-propargyl-uracil. Figure 2: Pd 0 -mediated prodrug-into-drug conversion assays in biocompatible environment. ( a ) Scanning electron microscope image of Pd 0 -resins at approximately 200 magnification. Scale bar, 50 μm. ( b ) Transmission electron microscope image of a Pd 0 -resin cross-section at approximately 190,000 magnification. Scale bar, 50 nm. ( c ) Pd 0 -mediated dealkylation of 5-fluorouracil (5FU) prodrugs under biocompatible conditions (37 °C, isotonic media and physiologic pH). ( d ) Representative HPLC traces of Pd 0 -mediated conversion of Pro-5FU into 5FU. Reaction crudes were analysed using an ultraviolet detector (280 nm) at t =0 h, t =6 h and t =24 h. Conversion studies were performed in triplicate. All-5FU , 1-allyl-5FU; Bn-5FU , 1-benzyl-5FU; Pro-5FU , 5-fluoro-1-propargyl-uracil. Full size image 1-Allyl-5FU ( All-5FU ), Pro-5FU and 1-benzyl-5FU ( Bn-5FU ; Fig. 2c ) were synthesized in a single step by reaction of 5FU with the corresponding alkyl bromide in the presence of 1,8-diazabicyclo[5.4.0]undec-7-ene. N -propargyl-2-pyridone ( 1a ) and N -propargyl-4-pyridone ( 1b ) were synthesized following the same procedure ( Supplementary Methods ). Cell-free Pd 0 -mediated prodrug-into-drug conversion To recreate a biocompatible scenario, reactions were carried out at 37 °C in an isotonic solution with a physiologic pH. Prodrugs (100 μM) and Pd 0 -resins (1 mg ml −1 , [Pd 0 ]=266 μM) were dispersed in PBS, incubated for 6–48 h and analysed by high-performance liquid chromatography (HPLC). Figure 2d shows Pro-5FU completely disappeared from the crude mixture after 24 h, with 5FU being the major reaction product. In accordance with previous observations [26] , mass spectrometry analysis of the reaction crude indicated the formation of nontoxic 1-hydroxyacetone—a natural lipid metabolite also known as acetol [29] —as a byproduct from the oxidative cleavage of the propargyl group ( Supplementary Fig. 2a,b ). In contrast, conversion analysis of All-5FU and Bn-5FU did not show substantial levels of 5FU after 48 h ( Supplementary Fig. 3a ). N -Depropargylation of Pro-5FU using sub-stoichiometric amounts of Pd 0 confirmed the catalytic nature of the reaction, albeit 72 h were required to achieve completion ( Supplementary Fig. 3b ). To determine whether Pro-5FU dealkylation is mediated by heterogeneous catalysis, Pd 0 -resins were incubated in PBS at 37 °C for 24 h, micro-filtered to eliminate solid contents and Pro-5FU added to the solid-free solution for additional 24 h incubation. HPLC analysis detected unreacted Pro-5FU as major mixture component and relatively small quantities of 5FU ( Supplementary Fig. 3c ), indicating that Pd 0 is in part released from the resins into the solution, although this amount contributes minimally to the reaction catalysis. Treatment of two additional N -propargylated heterocycles, N -propargyl-2-pyridone ( 1a ) and N -propargyl-4-pyridone ( 1b ), under the same conditions afforded the dealkylated derivatives in 24 h ( Supplementary Fig. 3d ). Pro-5FU bioorthogonality Based on the primary malignancies against which 5FU is currently prescribed [18] , [19] , colorectal HCT116 and pancreatic BxPC-3 cancer cell lines were chosen as models for antiproliferative and mechanism-of-action studies. To evaluate the efficacy of the masking strategy in suppressing 5FU cytotoxic properties, dose response studies were carried out with unmodified drug and Pro-5FU (0.01 μM to 1 mM). Cell viability was determined at day 5 using PrestoBlue reagent and analysed by spectrofluorometry to calculate EC 50 (5FU) values of 2 and 0.14 μM for HCT116 and BxPC-3 cells, respectively ( Supplementary Fig. 4a,b ). Notably, Pro-5FU displayed no cytotoxicity at any concentration used (EC 50 [ Pro-5FU ]/EC 50 [5FU]>500), proving the effectiveness of the deactivation strategy. To test whether Pro-5FU could be biotransformed into 5FU in cells with higher metabolic capacity, cell viability assays were carried out in liver HepG2 cells [30] . As shown in Supplementary Fig. 4c , although 5FU was significantly cytotoxic at low micromolar concentration (EC 50 =1.4 μM), Pro-5FU did not exhibit a toxic effect (EC 50 >1 mM), illustrating the high biochemical stability of the propargyl group to enzymatic cleavage. Because of the close structural similarities between Pro-5FU and 5FU, it was considered that the prodrug could function as a competitive inhibitor of the enzymatic routes followed by 5FU to generate its cytotoxic metabolites. This potential drawback of the prodrug strategy was ruled out by incubating 5FU with increasing concentrations of Pro-5FU up to a prodrug/drug ratio of 100:1, which exhibited no antagonistic effect ( Supplementary Fig. 5a,b ). In addition, dose response studies of 1-hydroxyacetone (main reaction byproduct) with HCT116 and BxPC-3 cancer cell lines showed no effect in cell viability ( Supplementary Fig. 5c,d ). Antiproliferative effect of Pro-5FU/Pd 0 -resin combination After assessing the catalyst concentration range tolerated by cells and optimal for catalysis ( Supplementary Fig. 6 ), 1 mg ml −1 (for HCT116) and 0.66 mg ml −1 (for BxPC-3) of Pd 0 -resins were used for the biological assays. Preliminary cell screening of palladium-mediated generation of 5FU from the three prodrugs confirmed that Pro-5FU /Pd 0 -resin combination was effective in producing a strong toxigenic effect ( Supplementary Fig. 7a,b ). Hence, a range of concentrations of Pro-5FU and Pd 0 -resins was incubated independently (negative controls) and in combination (BOOM conversion assay) to study cell proliferation in comparison to unmodified 5FU (positive control). As observed in Fig. 3a,b , the toxigenic effect generated by the prodrug/catalyst combination was comparable to 5FU cytotoxicity, exhibiting similar EC 50 values ( Supplementary Fig. 7c,d ). Independently incubated, neither the prodrug nor the palladium source exhibited antiproliferative activity. 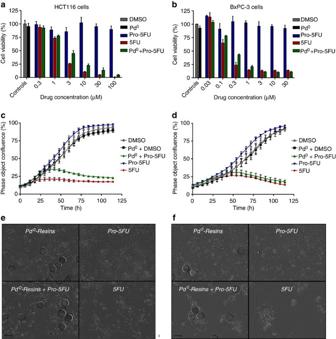Figure 3: Bioorthogonal generation of 5FU in cancer cell culture. Experiments: 0.1% (v/v) dimethylsulphoxide (DMSO, untreated cell control; in grey), Pd0-resins (negative control; in black); 0.01–100 μM of 5-fluoro-1-propargyl-uracil (Pro-5FU; negative controls; in blue); 0.01–100 μM of 5FU (positive controls; in red) and Pd0-resins+Pro-5FU(bioorthogonal organometallic conversion assay; in green). HCT116 and BxPC-3 cell studies are shown at the left and right side of the figure, respectively. Error bars represent ± standard deviation fromn=3. (a,b) Dose response study of cell viability after 5 days of treatment. (c,d) Real-time cell confluence study. Cell population was monitored for 5 days (120 h) using an IncuCyte ZOOM system in an incubator (5% CO2, 37 °C). Drug/prodrug concentrations: 100 μM, for HCT116 cells, and 30 μM, for BxPC-3 cells. (e,f) Phase-contrast images of cells after 4 days of treatment (96 h). Scale bar, 150 μm. Pd0-resins are identified as spheres of 150 μm (average diameter). Figure 3: Bioorthogonal generation of 5FU in cancer cell culture. Experiments: 0.1% (v/v) dimethylsulphoxide (DMSO, untreated cell control; in grey), Pd 0 -resins (negative control; in black); 0.01–100 μM of 5-fluoro-1-propargyl-uracil ( Pro-5FU ; negative controls; in blue); 0.01–100 μM of 5FU (positive controls; in red) and Pd 0 -resins+ Pro-5FU (bioorthogonal organometallic conversion assay; in green). HCT116 and BxPC-3 cell studies are shown at the left and right side of the figure, respectively. Error bars represent ± standard deviation from n =3. ( a , b ) Dose response study of cell viability after 5 days of treatment. ( c , d ) Real-time cell confluence study. Cell population was monitored for 5 days (120 h) using an IncuCyte ZOOM system in an incubator (5% CO 2 , 37 °C). Drug/prodrug concentrations: 100 μM, for HCT116 cells, and 30 μM, for BxPC-3 cells. ( e , f ) Phase-contrast images of cells after 4 days of treatment (96 h). Scale bar, 150 μm. Pd 0 -resins are identified as spheres of 150 μm (average diameter). Full size image Cytotoxic mode of action of Pro-5FU/Pd 0 -resin combination To study the phenotypic effect of the prodrug/catalyst system compared with 5FU, cell proliferation was monitored in real-time using an IncuCyte ZOOM microscope, which allows quantification of cell confluence as a function of time by image-based analysis. As shown in Fig. 3c,d , negative controls exhibited a standard growth curve, whereas the proliferation of cells treated with 5FU rapidly decreased after a few hours. Growth curves of HCT116 cells incubated with the Pd 0 -resin/ Pro-5FU combination showed two distinct phases: a regular increment for 24 h followed by a drastic fall to reach cytotoxic levels comparable to 5FU at day 5. In the case of BxPC-3 cells, population curves of cells incubated with either 5FU or the Pd 0 -resin/ Pro-5FU combination showed similar bell-shaped growth curves. As observed in Fig. 3e,f and Supplementary Movies 1 and 2 , treatment-induced changes in cell morphology indicate analogous antiproliferative/cell death induction between 5FU and the prodrug/catalyst system. To study these phenotypic responses at the molecular level, total expression and post-translational modifications of cancer relevant pathways were quantified using Zeptosens Reverse Phase Protein Microarray analysis [31] . Supplementary Fig. 8a shows that total and phosphorylated p53 (Ser15) were significantly upregulated in HCT116 cells at 24 h following exposure to Pro-5FU /Pd 0 -resin combination, which correlates with the response observed under 5FU treatment and the DNA damage response mechanism expected from this drug [32] . In contrast, no induction was observed in cells treated with either Pro-5FU or Pd 0 -resin on their own. These observations were corroborated by western blotting ( Supplementary Fig. 9 ). Pd 0 -Resin biocompatibility and catalytic activity in zebrafish The biocompatibility of the palladium-functionalized device in vivo was investigated by carefully introducing a single Pd 0 -resin in the yolk sac of zebrafish embryos 24 h after fertilization and monitoring their early development by phase contrast microscopy. As shown in Fig. 4a , zebrafish embryos containing a Pd 0 -resin (indicated with a red arrow) developed normally into the larval stage with no signs of toxicity or alteration of phenotype. 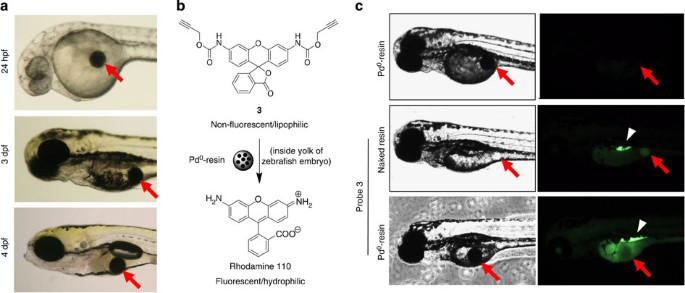Figure 4: Biocompatibility and catalytic activity of Pd0-resins in zebrafish embryos. (a) Images of a zebrafish embryo containing a Pd0-resin (red arrow) in the yolk sac at different stages of development. Twenty-four hours after fertilization (24 h.p.f.), a Pd0-resin was implanted in each embryo yolk (n=5), incubated at 28 °C and fish monitored for 4 days. Fish were imaged at 24 h.p.f., 3 days post fertilization (3 d.p.f.) and 4 d.p.f. (b) Palladium-mediated conversion of non-fluorescent lipophilic3into highly fluorescent hydrophilic rhodamine 110. (c)In vivocarbamate cleavage of3. One day after implantation, zebrafish embryos (n=5) containing a Pd0-resin (black colour) or a naked resin (white colour) in the yolk sac were incubated with3(5 μM) for 24 h at 31 °C. Subsequently, fish were imaged using confocal microscopy (Ex/Em: 488/521 nm). Pd0-resins and naked resin are indicated with red arrows. Fluorescently labelled gastrointestinal tract is indicated with a white arrow head. Figure 4: Biocompatibility and catalytic activity of Pd 0 -resins in zebrafish embryos. ( a ) Images of a zebrafish embryo containing a Pd 0 -resin (red arrow) in the yolk sac at different stages of development. Twenty-four hours after fertilization (24 h.p.f. ), a Pd 0 -resin was implanted in each embryo yolk ( n =5), incubated at 28 °C and fish monitored for 4 days. Fish were imaged at 24 h.p.f., 3 days post fertilization (3 d.p.f.) and 4 d.p.f. ( b ) Palladium-mediated conversion of non-fluorescent lipophilic 3 into highly fluorescent hydrophilic rhodamine 110. ( c ) In vivo carbamate cleavage of 3 . One day after implantation, zebrafish embryos ( n =5) containing a Pd 0 -resin (black colour) or a naked resin (white colour) in the yolk sac were incubated with 3 (5 μM) for 24 h at 31 °C. Subsequently, fish were imaged using confocal microscopy (Ex/Em: 488/521 nm). Pd 0 -resins and naked resin are indicated with red arrows. Fluorescently labelled gastrointestinal tract is indicated with a white arrow head. Full size image To study the catalytic functionality of the Pd 0 -resins in the zebrafish yolk, palladium-sensitive pro-fluorophore 3 ( Fig. 4b ) was prepared and incubated with zebrafish embryos containing either a non-functionalized resin (naked resin) or a Pd 0 -resin for 24 h. N , N′ -bis(propargyloxycarbonyl)-protected rhodamine 110 ( 3 ) was synthesized from rhodamine 110 chloride by reaction with propargyl chloroformate and triethylamine in dry dimethylformamide (DMF). The enhanced lipophilic properties of non-fluorescent probe 3 facilitated its diffusion across biological barriers. On the contrary, highly fluorescent rhodamine 110 generated upon propargylcarbamate cleavage was trapped in the physiological compartment where it was produced because of its high hydrophilicity, thus enabling the imaging of localized palladium-mediated catalysis [8] , [10] , [11] . As shown in Fig. 4c , a strong fluorescent signal was clearly observed from the area surrounding the Pd 0 -resin in the yolk sac (lower panel), confirming that the palladium-functionalized device is catalytically active in vivo . Concurrently, a strong fluorescent signal was also observed from the gastrointestinal system [33] , [34] in fish incubated with pro-fluorophore 3 regardless of the presence or absence of Pd 0 -resin ( Fig. 4c , pointed with white arrow heads, and Supplementary Fig. 10 ), suggesting that the N -propargyloxycarbonyl ( N -Poc) group is biochemically cleaved by digestive enzymes. Although 3 exhibited high sensitivity to palladium catalysis, it also displayed low chemical stability in the digestive system, indicating that N -Poc masked prodrugs could not be used via oral administration in a bioorthogonal strategy. For more than a decade [1] , [2] , [3] , the concept of bioorthogonal chemistry (understood as performing chemical reactions by artificial biologically inert means under biocompatible conditions) has inspired the search for novel biocompatible organic reactions and found a niche application as a labelling strategy to study biomolecules in their native state [1] , [2] , [3] , [4] , [5] , [35] . Indeed, bioorthogonal reactions have become particularly useful to study biological small molecules and macromolecules that cannot be monitored by genetically encoded reporters or antibodies (for example, lipids, glycans, and so on) both in cells and in vivo [4] , [35] . Although metal-free bioorthogonal reactions are considered optimal for living systems because of their biocompatibility, significant progress has been made in recent years in the development of cell-tolerated BOOM reactions [8] , [9] , [10] , [11] , [12] , [13] , [14] , [35] , [36] , opening up new avenues for the exploitation of the bioorthogonal paradigm. However, the potential of such selective processes in medicine is yet to be determined. Within an inclusive notion of bioorthogonality [5] , the clinical potential of bioorthogonal processes has only been explored to date with the photoinduced generation of cytotoxic reactive oxygen species through the use of a harmless visible light source and a non-toxic photosensitizer, which has become a valuable therapeutic option for local treatment of disease (so-called photodynamic therapy [37] ). In this line of reasoning, here we report a novel palladium-mediated N -dealkylation that takes place under biocompatible conditions and its application beyond the current scope of BOOM reactions: a highly efficient masking method that achieves complete elimination of 5FU cytotoxic activity, while enabling the bioorthogonal restoration of the drug's pharmacological properties by heterogeneous palladium chemistry in cell culture. In accordance with 5FU mode of action ( Fig. 1 ), modification of its N 1 position with each of the three alkyl groups investigated (allyl, propargyl and benzyl; Fig. 2c ) generates harmless prodrugs ( Supplementary Fig. 7a,b ), which demonstrates the low susceptibility of alkyl groups to cleavage by hydrolytic enzymes. However, under biocompatible conditions, only the propargyl group displays high sensitivity to Pd 0 -resins, thereby allowing the palladium-catalysed N-dealkylation of Pro-5FU at 37°C in PBS (isotonic, aqueous solution buffered at pH=7.4) within 24 h. Although the high stability of the benzyl moiety was anticipated because of the lack of an additional hydrogen source [20] , the drastic difference in Pd 0 sensitivity between Pro-5FU and All-5FU suggests that electronic and/or conformational aspects are critical for efficient metal coordination and cleavage ( Supplementary Fig. 2a ). To briefly examine the potential scope of the N -depropargylation process, N -propargyl-2-pyridone ( 1a ) and N -propargyl-4-pyridone ( 1b ) were synthesized and treated under the same conditions as Pro-5FU ( Supplementary Fig. 3d ). Dealkylated products were obtained within 24 h, indicating that this environmentally friendly methodology could be translated to other heterocyclic systems with lactam/lactim tautomery. Because of its implications for the bioorthogonal use of this novel masking/activation strategy, it is important to highlight that the palladium-mediated oxidative cleavage of the N -propargyl group in aqueous media results in the formation of non-toxic 1-hydroxyacetone [26] ( Supplementary Fig. 2b ). The generation of this natural compound [29] would minimize any local off-target effects caused by side products originated from the activation process itself. Our results show that, at the concentrations tested, neither the prodrug nor the palladium source exhibits antiproliferative activity in any of the cancer cell lines ( Fig. 3 ), thus validating the in vitro bioorthogonality of the materials. In contrast, the combined use of Pro-5FU and Pd 0 -resins led to a toxigenic effect comparable to 5FU antiproliferative activity, which demonstrates the in situ generation of 5FU. A variance in cytotoxicity was observed at several doses ( Fig. 3a,b ), which may be due to the time lag required for the BOOM reaction to take place and produce cytotoxic levels of drug. This difference was not significant in BxPC-3 cells at Pro-5FU doses higher than 1 μM ( Fig. 3b ), indicating that cytotoxic levels for this sensitive cell line are rapidly generated. Monitoring of HCT116 cell proliferation by time-lapse imaging allowed visualizing the slower antiproliferative effect led by the Pro-5FU /Pd 0 -resins combination (BOOM conversion assay) in comparison to unmodified 5FU ( Fig. 3c ). This result is in accordance with the time delay required to generate cytotoxic levels of drug for this cell line. Owing to the higher sensitivity of BxPC-3 cells to 5FU, both drug and the prodrug/catalyst combination experiments showed comparable bell-shaped population curves ( Fig. 3d ). In agreement with these observations, our immunoassay studies shows an analogous cell death induction mechanism between 5FU and the prodrug/catalyst system, corroborating that the cytotoxic activity generated by the prodrug/Pd 0 -resin combination is due to the BOOM synthesis of 5FU in cell culture. In conclusion, the development of a biochemically resistant palladium-labile 5FU precursor and an extracellular Pd 0 -functionalized device enabled the in vitro bioorthogonal transformation of a biologically inert substance into a cytotoxic agent. Although this novel prodrug strategy is yet to be tested in disease models in vivo , the robustness of the masking strategy, the biocompatibility of the dealkylation conditions and the innocuous reaction byproduct (natural product 1-hydroxyacetone [26] , [29] ) underline the therapeutic potential of this novel masking/activation approach. Finally, the biocompatibility and local catalytic activity exhibited by the Pd 0 -resin implanted within the zebrafish yolk supports the development of more comprehensive in vivo pharmacodynamics, pharmacokinetics and toxicity investigations in order to study the applicability and potential benefits of implementing a bioorthogonally activated prodrug approach. General methods Chemicals and solvents were purchased from Fisher Scientific, Sigma-Aldrich or VWR International Ltd. Nuclear magnetic resonance (NMR) spectra were recorded at ambient temperature on a 500-MHz Bruker Avance III spectrometer (Bruker). Chemical shifts are reported in parts per million (p.p.m.) relative to the solvent peak. Rf values were determined on Merck TLC Silica gel 60 F254 plates (Merck) under a 254-nm ultraviolet source. Purification of compounds was carried out via manual flash column chromatography using commercially available silica gel (220–440 mesh, Sigma-Aldrich). Cell lines were grown in culture media supplemented with serum (10% fetal bovine serum) and L -glutamine (2 mM) and incubated in a Heracell 240i tissue culture incubator at 37 °C and 5% CO 2 . Human colorectal carcinoma HCT116 cells (a kind gift from Dr Van Schaeybroeck) were cultured in Dulbecco's Modified Eagle Media (DMEM). Human pancreas adenocarcinoma BxPC-3 cells (a kind gift from Dr Mark Duxbury) were cultured in Roswell Park Memorial Institute media. Human hepatocyte carcinoma HepG2 cells were obtained from Sigma-Aldrich and cultured in DMEM. Synthesis and characterization of Pd 0 -resins NovaSyn TG amino resin HL (1,000 mg, 0.39 mmol NH 2 per g) and palladium acetate (263 mg, 1.17 mmol) were added into a 25 ml Biotage microwave vial (Biotage) with toluene (10 ml) and heated to 80 °C under stirring for 10 min. The mixture was then stirred at room temperature for 2 h and the resins subsequently filtered and washed with dichloromethane (5 × 20 ml) and methanol (5 × 20 ml). Resins were dispersed in 10% hydrazine monohydrate in methanol (10 ml) and stirred at room temperature for 25 min. The resins were then filtered and washed with methanol (5 × 20 ml) and dichloromethane (5 × 20 ml). Resins were added to a solution of Fmoc-Glu(OH)-OH (216 mg, 0.59 mmol), Oxyma (166 mg, 1.17 mmol), N , N ′-diisopropylcarbodiimide (DIC) (148 mg, 1.17 mmol) and DCM/DMF (2:1, 9 ml) and stirred for 2 h at room temperature. The resins were filtered and washed with dichloromethane (5 × 20 ml), methanol (5 × 20 ml) and H 2 O (5 × 20 ml) and dried in an oven at 40 °C for 3 days. Complete coupling was verified by the ninhydrin test after the last methanol wash. Scanning electron microscope/transmission electron microscope images and Pd 0 quantification (by inductively coupled plasma-optical emission spectrometry) were carried out as previously described [8] . Resins were characterized using X-ray difractometry (Bruker D2 PHASER with LYNXEYE detector (Bruker), Cu radiation source at 30 kV, 10 mA and a Ni filtre) before and after Pd 0 -functionalization. Without any extra preparation or post-processing, samples were mounted on a 1 inch diameter standard holder. The phase constituents were identified as per Supplementary Fig. 1c . Synthesis and characterization of 5FU prodrugs 5FU (200 mg, 1.54 mmol) and 1,8-diazabicyclo[5.4.0]undec-7-ene (269 μl, 1.80 mmol) were dissolved in dry DMF (2 ml) under N 2 atmosphere and cooled to 4 °C. Either allyl, propargyl or benzyl bromide (1.54 mmol) were dissolved in dry DMF (0.5 ml). The solution was added dropwise to the mixture and the resulting mixture stirred at room temperature overnight. Solvents were then removed under reduced pressure and the crude purified via flash chromatography (3% MeOH in DCM). 1-Allyl-5FU ( All-5FU ): colourless solid, 80 mg (31% yield); Rf=0.5 (6% MeOH in DCM); 1 H NMR (500 MHz, dimethylsulphoxide (DMSO)- d 6 ) δ =11.80 (br s, 1H, N H ), 8.01 (d, J (HH)=6.7 Hz, 1H, Ar H ), 5.88 (ddt, J (HH)=17.0, J (HH)=10.5 Hz, J (HH)=5.5 Hz, 1H, N–CH 2 –C H ), 5.19 (m, 2H, CH 2 –CH=C H 2 ), 4.24 (d, J (HH)=5.3 Hz, 2H, N–C H 2 –CH); 13 C NMR (126 MHz, DMSO) δ =157.45 (d, J (CF)=25.5 Hz, C), 149.46 (C), 139.68 (d, J (CF)=229.5 Hz, C), 132.63 (CH), 129.79 (d, J (CF)=33.0 Hz, CH), 117.64 (CH 2 ), 49.34 (CH 2 ); high-resolution mass spectrometry (HRMS) fast atom bombardment (FAB) ( m/z ): [M] + calcd for C 7 H 7 O 2 N 2 F, 170.0486; found, 170.0489. Pro-5FU : colourless solid, 104 mg (40% yield); Rf=0.35 (6% MeOH in DCM); 1 H NMR (500 MHz, DMSO- d 6 ) δ =11.91 (br s, 1H, N H ), 8.13 (d, J (HH)=5.0 Hz, 1H, Ar H ), 4.46 (d, J (HH)=2.5 Hz, 2H, N–C H 2 –C), 3.44 (t, J (HH)=2.5 Hz, 1H, C≡C H ); 13 C NMR (126 MHz, DMSO) δ =157.35 (d, J (CF)=26.0 Hz, C), 149.11 (C), 139.80 (d, J (CF)=230.5 Hz, C), 128.95 (d, J (CF)=34.0 Hz, CH), 78.40 (C), 76.15 (CH), 37.00 (CH 2 ); HRMS (FAB) ( m/z ): [M] + calcd for C 7 H 5 O 2 N 2 F, 168.0332; found, 168.0330. 1-Benzyl-5FU ( Bn-5FU ): pale yellow solid, 133 mg (38% yield); Rf=0.44 (6% MeOH in DCM); 1 H NMR (500 MHz, DMSO- d 6 ) δ =11.86 (br s, 1H, N H ), 8.22 (d, J (HH)=6.7 Hz, 1H, Ar H ), 7.39–7.28 (m, 5H, Ar H ), 4.83 (s, 2H, N–C H 2 –Ph); 13 C NMR (126 MHz, DMSO- d 6 ) δ =157.42 (d, J (CF)=25.5 Hz, C), 149.68 (C), 139.62 (d, J (CF)=228.0 Hz, C), 136.52 (C), 130.08 (d, J (CF)=33.5 Hz, CH), 128.67 (CH), 127.75 (CH), 127.49 (CH), 50.63 (CH 2 ); HRMS (FAB) ( m/z ): [M] + calcd for C 11 H 9 O 2 N 2 F, 220.0643; found, 220.0643. Synthesis and characterization of probe 3 Rhodamine 110 chloride (250 mg, 0.68 mmol) was dissolved in dry DMF (4 ml) under nitrogen atmosphere. Separately, propargyl chloroformate (273 μl, 2.80 mmol) and triethylamine (488 μl, 3.50 mmol) were added dropwise to the mixture. The reaction mixture was stirred at room temperature for 48 h, solvents removed in vacuo and the resulting crude re-suspended in 25% isopropanol in DCM (20 ml) and washed with H 2 O. The aqueous layer was then washed five times with 25% isopropanol in DCM (20 ml). The combined organic layers were dried over anhydrous MgSO 4 , the solids filtered off and concentrated in vacuo . Crude was purified via flash chromatography (hexane/ethyl acetate 2:1) and yielded bis- N , N′ -propargyloxycarbonyl-rhodamine 110 ( 3 ) as a white solid (67 mg, 20%). Rf=0.13 (hexane/ethyl acetate 2:1); 1 H NMR (500 MHz, CD 3 OD) δ =8.02 (d, J (HH)=7.5 Hz, 1H, Ar H ), 7.77 (td, J (HH)=7.5 Hz, 1.1, 1H, Ar H ), 7.71 (td, J (HH)=7.5 Hz, 0.9, 1H, Ar H ), 7.61 (d, J (HH)=2.0 Hz, 2H, Ar H ), 7.21 (d, J (HH)=7.6, 1H, Ar H ), 7.08 (dd, J (HH)=8.5 Hz, 2.2, 2H, Ar H ), 6.68 (d, J (HH)=8.5 Hz, 2H, Ar H ), 4.78 (d, J (HH)=2.4 Hz, 4H, C H 2 –C≡CH), 2.94 (t, J (HH)=2.4 Hz, 2H, C≡C H ); 13 C NMR (126 MHz, MeOD) δ =171.35 (C), 154.59 (C), 154.43 (C), 153.18 (C), 142.65 (C), 136.74 (CH), 131.27 (CH), 129.47 (CH), 127.76 (C), 125.89 (CH), 125.19 (CH), 115.60 (CH), 114.42 (C), 107.04 (CH), 84.48 (C), 79.08 (C), 76.22 (C), 53.40 (CH 2 ); mass spectrometry (electrospray ionization) ( m/z ): 495.2 [M+H] + . Pd 0 -mediated prodrug dealkylation in biocompatible environ All-5FU , Pro-5FU and Bn-5FU (100 μM) were dissolved in PBS (1 ml) with 1 mg of Pd 0 -resins and shaken at 1,400 r.p.m. and 37 °C in a Thermomixer. Reaction crudes were monitored at 0, 6, 24 and 48 h by analytical HPLC (Agilent) using the ultraviolet detector at 280 nm to avoid the detection of PBS salts. Eluent A: water and formic acid (0.1%); eluent B: acetonitrile, formic acid (0.1%); A/B=95:5 to 5:95 in 3 min, isocratic 1 min, 5:95 to 95:5 in 1 min, isocratic 1 min. Catalytic conversion assay: Pro-5FU in 0.1% (v/v) DMSO was dissolved in PBS (1 ml) with Pd 0 -resins (1 mg ml −1 , [Pd 0 ]~266 μM) to reach a final Pro-5FU concentration 300 μM and incubated for 24, 48, 72 h at 37 °C. Pro-5FU presence was monitored by HPLC. For the heterogeneous catalysis assay, Pd 0 -resins (2 mg) were dispersed into a PBS solution (2 ml) and incubated for 24 h at 37 °C. The mixture was filtrated using a Millipore microfiltre (0.22 μm, Millipore) and, subsequently, Pro-5FU added to the mixture (final concentration=100 μM). The reaction mixture was incubated for additional 24 h and analysed by HPLC (ultraviolet detector at 280 nm). Cell viability studies of 5FU versus Pro-5FU Cells were seeded in a 96-well plate format at the appropriate cell concentration (3,000 cells per well for HCT116 and BxPC-3 cells, and 4,000 cells per well for HepG2 cells) and incubated for 48 h before treatment. Each well was then replaced with fresh media containing 5FU (0.01 μM to 1 mM) with DMSO (0.1% v/v); or Pro-5FU (0.01 μM to 1 mM) with DMSO (0.1% v/v) and incubated for 5 days. Untreated cells were incubated with DMSO (0.1% v/v). PrestoBlue cell viability reagent (10% v/v) was added to each well and the plate incubated for 45 min. Fluorescence emission was detected using a PerkinElmer EnVision 2101 multilabel reader (Perkin Elmer; excitation filtre at 540 nm and emissions filtre at 590 nm). All conditions were normalized to the untreated cells (100%) and curves fitted using GraphPad Prism using a sigmoidal variable slope curve. Pd 0 -mediated dealkylation of Pro-5FU in cell culture HCT116 and BxPC-3 cells were seeded in a 96-well plate format with a density of 3,000 cells per well and incubated for 48 h before treatment. Each well was then replaced with fresh media containing: Pd 0 -resins (0.67 or 1 mg ml −1 for BxPC-3 or HCT116, respectively) with DMSO (0.1% v/v); Pro-5FU (0.01–100 μM) with DMSO (0.1%, v/v); 5FU (0.01 μM to 1 mM) with DMSO (0.1%, v/v) or combination of Pd 0 -resin+ Pro-5FU (0.01–100 μM) with DMSO (0.1%, v/v). Untreated cells were incubated with DMSO (0.1% v/v). For the cell viability assay, cells were incubated with drugs for 5 days. PrestoBlue cell viability reagent (10% v/v) was added to each well and the plate incubated for 45 min. Fluorescence emission was detected and results normalized as described above. For the time lapse imaging study, cell growth studies were carried out at a single dose of 5FU or Pro-5FU (100 μM for HCT116 and 30 μM for BxPC-3). Each well was imaged every 2 h over 5 days under standard incubation conditions using an IncuCyte ZOOM microscope (placed inside the incubator). Imaged-based analysis of cell confluence and Supplementary Movies 1 and 2 were carried out using the IncuCyte software. Reverse phase protein array analysis Cells were plated in a 6-well plate at a density of 480,000 cells per well and incubated for 48 h. Before adding the prodrug to the HCT116 cells, Pro-5FU (100 μM) and Pd 0 -resins (1 mg ml −1 ) were incubated in media at 37 °C for 24 h to overcome the time delay required to convert Pro-5FU into 5FU, which was seen to have a relevant effect in this cell type. This pre-incubation procedure was not carried out for the study with BxPC-3 cells (30 μM). Pd 0 resin/ Pro-5FU combination and the controls (as before, untreated cells; Pd 0 -resins; Pro-5FU and 5FU) were incubated with each cell line for 6 and 24 h. Afterwards, the cells were washed with PBS (2 × 3 ml) and lysed with Zeptosens CLB1 lysis buffer (90 μl, Zeptosens). Samples were analysed by Zeptosens RPPA (Zeptosens) as previously described [31] using the following specific conditions. Tumour cell lysates were normalized to a uniform protein concentration with spotting buffer CSBL1 (Zeptosens-Bayer) before preparing a final fourfold concentration series of 0.2, 0.15, 0.1 and 0.05 mg ml −1 . The diluted concentration series of each sample was printed onto Zeptosens protein microarray chips (ZeptoChip, Zeptosens-Bayer) under environmentally controlled conditions (constant 50% humidity and 14 °C temperature) using a non-contact printer (Nanoplotter 2.1e, GeSiM). A single 400 Pico litre droplet of each lysate concentration was deposited onto the Zeptosens chip (thus representing four spots per each biological replicate). A reference grid of Alexa Fluor-647 conjugate BSA consisting of 4 column × 22 rows was spotted onto each sub-array. Each sample concentration series were spotted in between reference columns. After array printing, the arrays were blocked with an aerosol of BSA solution using a custom designed nebulizer device (ZeptoFOG, Zeptosen-Bayer) for 1 h. The protein array chips were subsequently washed in double-distilled H 2 O and dried before performing a dual antibody immunoassay comprising of a 24-h incubation of primary antibody (the library of primary antibodies used is in Supplementary Table 1 and were purchased from Cell Signaling Technologies) followed by 2.5 h incubation with secondary Alexa Fluor-conjugated antibody detection reagent (anti-rabbit A647 Fab; Invitrogen). Following secondary antibody incubation and a final wash step in BSA solution, the immunostained arrays were imaged using the ZeptoREADER instrument (Zeptosens-Bayer). For each sub-array, five separate images were acquired using different exposure times ranging from 0.5 to 10 s. Microarray images representing the longest exposure without saturation of fluorescent signal detection were automatically selected for analysis using the ZeptoView 3.1 software (Zeptosens-Bayer). A weighted linear fit through the fourfold concentration series was used to calculate relative fluorescence intensity (RFI) value for each sample replicate. Local normalization of sample signal to the reference BSA grid was used to compensate for any intra- or inter-array/chip variation. Local normalized RFI values were used for all subsequent analysis. Abundance levels of total p53 protein, phosphorylated p53 (Serine 15) and phosphorylated Akt (Ser 473) were plotted as RFI data calculated by the ZeptoView 3.1 software. Western blot analysis Cell lysates for HCT116 and BxPC-3 cells were prepared as described above for Zeptosens analysis. Protein samples (35 μg) and SeeBlue Plus2 Pre-Stained Standard (7.5 μg) were separated by SDS-PAGE (Bio-Rad, 4–15% gels) and transferred to PVDF membranes (GE). Western blotting was performed using rabbit monoclonal antibodies against human p53 and Phospho-p53 (Ser 15) (1:1,000 for each one, Cell Signaling Technologies, cat. no. 9282 and 9284, respectively) at 4 °C overnight. This was followed by 1 h incubation at room temperature with secondary horseradish peroxidase (HRP)-linked antibody (1:10,000, anti-rabbit IgG, Sigma). The loading control, actin, was detected using a mouse monoclonal antibody (1:40,000, Calbiochem, cat. no. CP01) followed by a secondary HRP-linked antibody treatment (1:40,000, anti-mouse IgM, Calbiochem). HRP was detected by addition of POD ECL (Roche) and bands visualized using a ChemiDoc MP Imager (Bio-Rad). Zebrafish studies For the biocompatability assay, wild-type zebrafish embryos were collected from AB-TPL breeding pairs and reared at 28 °C in E3 embryo medium. Twenty-four hours post fertilization, embryos were treated with tricaine (anesthetic) and pierced in the yolk with a fine needle. Either a naked resin or a Pd 0 -resin was then rapidly inserted into the yolk opening to minimize loss of yolk. Embryos that lost significant yolk in the procedure were removed from the experiment. Embryos were then gently transferred to fresh E3 medium ( n =5), returned to 28 °C and monitored over 3 days by microscopy. For the catalytic activity assay, either a naked resin or a Pd 0 -resin was implanted in 24 h.p.f. zebrafish embryos ( n =5) following the above procedure and gently transferred to fresh E3 medium. Embryos were incubated for 24 h at 28 °C to ensure the yolk wound was closed. Embryos that lost significant yolk in the procedure were removed from the experiment. 3 was added to the embryo medium (final concentration 5 μM) and fish incubated for additional 24 h at 31 °C to increment the probe activation rate. Fish were imaged using fluorescent microscopy (Olympus Scan-R, Olympus). It is important to note that the zebrafish embryos looked older than developmental 3 d.p.f., probably due to the increased incubation temperature (31°C). Experiments were repeated three times. Zebrafish husbandry and experiments were performed under Home Office License in compliance with the Animals (Scientific Procedures) Act 1986, and approved by the University of Edinburgh Ethics Committee. How to cite this article: Weiss, J. T. et al. Extracellular palladium-catalysed dealkylation of 5-fluoro-1-propargyl-uracil as a bioorthogonally activated prodrug approach. Nat. Commun. 5:3277 doi: 10.1038/ncomms4277 (2014).